Holocene winter climate variability in mid-latitude western North America Water resources in western North America depend on winter precipitation, yet our knowledge of its sensitivity to climate change remains limited. Similarly, understanding the potential for future loss of winter snow pack requires a longer perspective on natural climate variability. Here we use stable isotopes from a speleothem in southwestern Oregon to reconstruct winter climate change for much of the past 13,000 years. We find that on millennial time scales there were abrupt transitions between warm-dry and cold-wet regimes. Temperature and precipitation changes on multi-decadal to century timescales are consistent with ocean-atmosphere interactions that arise from mechanisms similar to the Pacific Decadal Oscillation. Extreme cold-wet and warm-dry events that punctuated the Holocene appear to be sensitive to solar forcing, possibly through the influence of the equatorial Pacific on the winter storm tracks reaching the US Pacific Northwest region. Long, high-resolution and well-dated paleoclimate data sets that capture regional patterns and timing of climate change extend instrumental records, thus increasing our understanding of the full range of natural climate variability and its sensitivity to potential forcings. Many high-resolution paleoclimate records, such as those based on tree rings, are biased towards recording climate conditions during the summer season, the critical period for plant growth. There is less information available, however, for winter season conditions, which in regions such as western North America are critical for determining water resources. Regional climate in the Pacific Northwest is strongly influenced by atmosphere–ocean interactions that originate in the Pacific Ocean on seasonal, interannual, decadal and presumably also longer timescales. Strong seasonality develops from contrasts in ocean–continent heating, with relatively warm and dry summers associated with the northward migration of the Pacific subtropical high, and cool and wet winters associated with an intensification of the Aleutian low. Southward displacement of the Pacific subtropical high-pressure cell by the Aleutian low-pressure system brings a predominance of southwesterly winds and abundant precipitation during winter months. The North Pacific has a high frequency of winter (December-February) storms particularly north of 40°N where cyclone densities exceed 2 × 10 −3 (deg. lat.) −2 (ref. 1 ). The climate in Oregon is also sensitive to interannual and decadal changes associated with the El Niño-Southern Oscillation (ENSO) and Pacific Decadal Oscillation (PDO), respectively, that are particularly well expressed during the winter season [2] , [3] , modulating seasonal contrasts in temperature and precipitation ( Fig. 1 ). Approximately 85% of the mean annual precipitation (1,600 mm) at Oregon Caves National Monument (OCNM) falls between November and April. 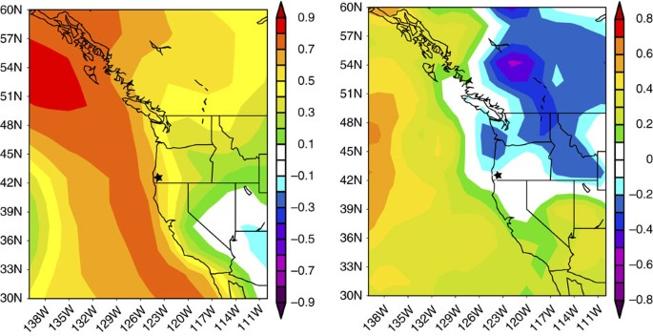Figure 1: Map of western North America. NCEP/NCAR reanalysis showing the correlation between surface air temperature (left) and precipitation rate (right) with the PDO index during the cool season (November–March) in the Pacific Northwest for the period 1949–2006. Location of OCNM is marked by a star. Figure 1: Map of western North America. NCEP/NCAR reanalysis showing the correlation between surface air temperature (left) and precipitation rate (right) with the PDO index during the cool season (November–March) in the Pacific Northwest for the period 1949–2006. Location of OCNM is marked by a star. Full size image The hydrologic system at OCNM responds rapidly to these seasonal changes in precipitation. Observations at the cave show that after summer desiccation, dripwater is initiated within a month of the onset of the winter rainy season, and ends in the early summer after runoff of snowmelt. Almost all stalagmite growth thus occurs between November and June, making this site ideally suited for documenting long-term variations in winter storm tracks that bring precipitation into much of western North America [4] . Here we reconstruct winter climate variability in southwestern Oregon, USA, for much of the past 13,000 years (13 ka) at decadal and longer scales based on a U-Th-dated high-resolution stable isotope record captured in a stalagmite from OCNM (42°05′ N, 123°25′ W, ~1,200 m above sea level, Fig. 1 ). We use oxygen (δ 18 O) and carbon (δ 13 C) stable isotopes from stalagmite OCNM02-1 [5] and find that long-term changes in δ 18 O track orbitally modulated insolation, consistent with sensitivity of winter temperature to seasonal radiative forcing in models that include oceanic processes. At millennial timescales, we identify abrupt shifts between warm-dry versus cold-wet regimes, indicating large natural climate variability. Extreme cold-wet events that punctuated the Holocene, with a mean recurrence time of 1.0±0.4 ka and persistence of 100s of years, coincide with episodes of low global 10 Be flux and 14 C production, implying a sensitive response to solar forcing plausibly through the influence of the equatorial Pacific on the US Pacific Northwest winter storm tracks. Multi-decadal and centennial variability is consistent with ocean–atmosphere interactions similar to the PDO. Stable isotope interpretation Modern rainfall δ 18 O at the site correlates with monthly temperature ( r 2 =0.65) and precipitation amount effects are relatively small [4] . When combined with the counteracting effects of cave temperature on isotopic equilibrium in calcitic speleothems [6] , the net scaling of speleothem δ 18 O to surface air temperature is 0.7‰ per °C. Support for a precipitation–temperature control on speleothem δ 18 O at OCNM comes from a previous study of an older segment of the same stalagmite [7] , in which lower δ 18 O values document a clear signal of the Younger Dryas cold event ( Fig. 2b ), which is also expressed in nearby marine [8] ( Fig. 2a ) and pollen [9] records. 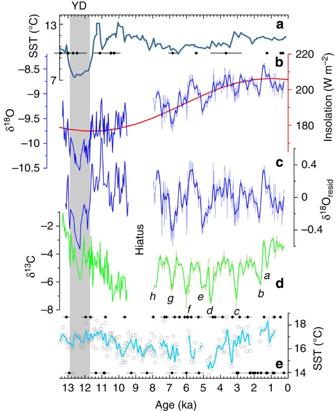Figure 2: Palaeoclimate timeseries. (a) Alkenone-derived SSTs off the coast of northern California8. Symbols below time series represent the calibrated14C ages with 1σ uncertainties. (b) The δ18O record at OCNM (blue) and November solar insolation18at 42°N (red). (c) The δ18O record at OCNM with the insolation trend removed. In bothb,c, the high-resolution record is shown with light blue lines, whereas the thick blue lines represent the smoothed time series (50-year resolution). (d) The δ13C record at OCNM. The high-resolution record is shown with a light green line, whereas the thick green line represents the smoothed time series (50-year resolution). Symbols below δ13C time series represent the U-Th ages with 2σ uncertainties. Pronounced negative excursions in the δ13C record are identified as events a-h. (e) Mg/Ca-derived SST in the Soledad Basin35. The grey circles represent the Mg/Ca data, and the blue line shows the smoothed record at a 50-year resolution. Symbols below time series represent the calibrated14C ages with 1σ uncertainties. The grey vertical bar marks the Younger Dryas (YD) cold event52. Figure 2: Palaeoclimate timeseries. ( a ) Alkenone-derived SSTs off the coast of northern California [8] . Symbols below time series represent the calibrated 14 C ages with 1σ uncertainties. ( b ) The δ 18 O record at OCNM (blue) and November solar insolation [18] at 42°N (red). ( c ) The δ 18 O record at OCNM with the insolation trend removed. In both b , c , the high-resolution record is shown with light blue lines, whereas the thick blue lines represent the smoothed time series (50-year resolution). ( d ) The δ 13 C record at OCNM. The high-resolution record is shown with a light green line, whereas the thick green line represents the smoothed time series (50-year resolution). Symbols below δ 13 C time series represent the U-Th ages with 2σ uncertainties. Pronounced negative excursions in the δ 13 C record are identified as events a-h. ( e ) Mg/Ca-derived SST in the Soledad Basin [35] . The grey circles represent the Mg/Ca data, and the blue line shows the smoothed record at a 50-year resolution. Symbols below time series represent the calibrated 14 C ages with 1σ uncertainties. The grey vertical bar marks the Younger Dryas (YD) cold event [52] . Full size image The δ 13 C of OCNM speleothem calcite records the influence of precipitation and vegetation on the dissolved inorganic carbon of dripwaters [10] . An increase in precipitation may cause lower speleothem δ 13 C directly through its effects on cave hydrology [11] , [12] and indirectly through its influence on surface biomass [13] . Changes in plant photosynthetic pathways [14] (C 3 versus C 4 plants) can also affect speleothem δ 13 C, but pollen data [15] show that C 3 vegetation has dominated the local biomass over the last 10 ka, suggesting that this effect is not important at OCNM. We thus use speleothem δ 13 C at OCNM to infer relative variations in precipitation and its associated effects on biomass and soil in the cave’s water recharge zone, consistent with the results of δ 13 C modelling in speleothems from a cave site 500 km to the south, which has a similar Mediterranean-type climate and bedrock type [16] . Age model We derive an age model and its uncertainties for the stalagmite from 29 high-precision U-Th dates ( Supplementary Fig. S1 and Supplementary Table S1 ) using Markov Chain Monte–Carlo sampling and Bayesian statistics implemented in the OxCal 4.1 program [17] . We take into account possible uncertainties in transferring the depth scale of the U-Th ages to the depth scale of the isotope time series, and together with the U-Th age uncertainties we estimate changes in growth rate using a Monte–Carlo approach ( Fig. 3a ) after excluding the options that have negative growth rate. A high-resolution stable isotope record spans the interval from 0.2 to 7.9 ka ( Fig. 2 ); here speleothem growth rates range from 8.1 to 60 μm year −1 ( Fig. 3a ), and an effective block-average sampling interval of 3 years. A hiatus in speleothem growth rate extending from 8.0 to ~9.5 ka is visible as a dark layer that contains detrital material ( Supplementary Fig. S1 ). We combine this record with a previously published lower resolution record from the same stalagmite [7] that covers the interval from ~13.3 ka to the start of the hiatus at 9.5 ka ( Fig. 2 ). 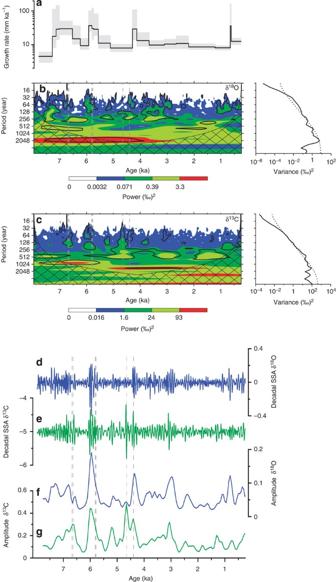Figure 3: Timeseries characterization. (a) Growth rates for OCNM02-1 speleothem with the Monte–Carlo uncertainty envelope shown in grey. (b) Morlet wavelet and global wavelet spectrum for OCNM δ18O. (c) Morlet wavelet and global wavelet spectrum for OCNM δ13C. The areas on the wavelets outlined with black lines are significant at the 90% level, and the cone of influence is shown with hashed lines. Dashed lines in the global wavelet spectrum represent the 90% confidence level. SSA-extracted decadal variability at OCNM for δ18O (d) and δ13C (e) together with amplitude modulation of decadal variability for δ18O (f) and δ13C (g). Dashed vertical grey lines represent the position of changes in isotope sampling track. Figure 3: Timeseries characterization. ( a ) Growth rates for OCNM02-1 speleothem with the Monte–Carlo uncertainty envelope shown in grey. ( b ) Morlet wavelet and global wavelet spectrum for OCNM δ 18 O. ( c ) Morlet wavelet and global wavelet spectrum for OCNM δ 13 C. The areas on the wavelets outlined with black lines are significant at the 90% level, and the cone of influence is shown with hashed lines. Dashed lines in the global wavelet spectrum represent the 90% confidence level. SSA-extracted decadal variability at OCNM for δ 18 O ( d ) and δ 13 C ( e ) together with amplitude modulation of decadal variability for δ 18 O ( f ) and δ 13 C ( g ). Dashed vertical grey lines represent the position of changes in isotope sampling track. Full size image Speleothem stable isotope record The average δ 18 O value of the stalagmite for the most recent millennium (−8.81±0.14‰ s.d., n =251) is in good agreement with δ 18 O values measured on two active soda-straw stalactites sampled in 2006 (−8.77 and −8.87‰), implying that modern conditions are within the range of recent preanthropogenic variability. After accounting for the effect of small changes in global seawater δ 18 O in the early Holocene [7] , the full Holocene record reveals a long-term trend in δ 18 O that increases from −9.69±0.25‰ s.d. ( n =27) in the early Holocene (11.5–10.5 ka) to −8.81±0.14‰ s.d. ( n =251) for the most recent millennium ( Fig. 2b ). This trend closely parallels the orbitally forced increase in winter insolation through the Holocene. Although the differences between the amplitude of orbitally modulated solar insolation change during individual winter months are small [18] , an empirical best fit to the speleothem δ 18 O data is given by November insolation [18] ( Fig. 2b ). We speculate that this finding reflects the fact that November represents the modern transition from the dry season to the rainy season [19] , and thus influences the length of time that the speleothem accumulates each year. On the basis of our derived local δ 18 O:temperature relation, we infer a ~1.0 °C winter warming through the Holocene, equivalent to a sensitivity to November insolation forcing of 0.07 °C per W m −2 . This sensitivity estimate is a lower limit; a disequilibrium (that is, lagging) response to seasonal insolation earlier in the year would imply a greater equilibrium sensitivity. Furthermore, if cool-wet years were associated with extension of the rainy season into the warmer summer months, apparent winter temperature change would likely be underestimated by δ 18 O. The observed long-term trend and sensitivity are consistent with the results for this region in transient simulations with global coupled atmosphere–ocean models forced by insolation [20] but are of opposite sign to winter climate anomalies produced in a regional atmosphere climate model, which held ocean temperatures at modern values [19] , pointing to the importance of oceanic processes for the winter climate in this area. Superimposed on the long-term warming trend is persistent multi-decadal to millennial variability characterized by abrupt transitions between warm (high-δ 18 O) and cold (low-δ 18 O) states ( Fig. 2c ). This pattern repeats with roughly constant amplitude through the Holocene increase in November insolation, implying that its underlying cause is insensitive to changes in the background climate state associated with such seasonal insolation forcing. Particularly noteworthy are distinct millennial-scale fluctuations with amplitudes of ~0.8‰, as large as the long-term Holocene increase in δ 18 O, that are punctuated by abrupt century-scale cool intervals centred near 12.3, 10.4, 7.4, 6.8, 6.0, 5.0, 3.1, 1.7 and 0.6 ka ( Fig. 2b ). Unlike the δ 18 O record, there is no significant long-term trend in the δ 13 C time series ( Fig. 2d ). The two isotope records are otherwise similar in their multi-decadal to millennial-scale variability, with all but one of the eight particularly pronounced and abrupt δ 13 C depletion events of as much as 4‰ (labelled a–h in Fig. 2 ) being nearly synchronous with the largest cool events seen in the δ 18 O record. During the ~1,200-year-long Younger Dryas interval, a significant δ 13 C and δ 18 O depletion event occurs as a ~400-year excursion from ~12.5–12.1 ka ( Fig. 2c ). This excursion within the longer Younger Dryas cool event may be analogous to the Holocene cold-wet excursions, implying that millennial-scale variability may occur here independently of the background climatic state, and suggesting the presence of an independent external forcing mechanism. One of the prominent features in the δ 13 C record is the shift towards more positive values that occurs at ~1.6 ka. This change coincides with the timing of increased ENSO variability, as suggested by both proxy and modelling studies [21] , [22] , [23] as part of a change in tropical Pacific dynamics during the late Holocene [24] . More frequent/stronger El Niño events would likely correspond to a warmer/drier climate at OCNM, leading to more positive δ 13 C values modulated by changes in organic productivity in the overlying forest and soil system. During this interval, the Little Ice Age (LIA, 1,450–1,850 Common Era (CE)) was characterized by overall lower δ 13 C values compared with the Medieval Climate Anomaly (MCA, 1,000–1,400 CE), a difference that is statistically significant (see Methods) and consistent with a wetter winter period. Given the observed long-term increasing trend in δ 18 O and its plausible relation to seasonal insolation forcing, the absence of a similar δ 13 C trend implies no significant temperature control on environmental factors influencing δ 13 C, which we infer to be ultimately linked to precipitation. In particular, if such a temperature control existed, δ 13 C would mimic δ 18 O on all time scales, not just at higher frequencies. We thus infer that precipitation amount and biomass at OCNM were largely insensitive to long-term seasonal insolation forcing during the Holocene. A Morlet wavelet transform provides insight into the non-stationary nature of the variability in the data [25] . Our analysis is limited to the interval <8 ka (that is, younger than the hiatus, where sampling resolution was highest). The long-term trend in δ 18 O, attributed to solar insolation, was removed before analysis ( Fig. 2c ). For δ 18 O, a ~2,000-year cycle is statistically significant (90% confidence) in the early-mid Holocene (~7.5–4 ka) but is not distinguishable from red noise in the full record. Significant intervals of multi-decadal and multi-centennial variability come and go intermittently ( Fig. 3b ). For δ 13 C, the wavelet reveals a statistically significant ~1,500-year cycle during the middle-late Holocene (90% confidence, but not significant relative to stochastic red noise over the full record) and a ~500-year cycle (statistically significant above stochastic noise, 90% confidence) through most of the Holocene ( Fig. 3c ). Similar centennial-to-millennial-scale variability was also identified in the western North Pacific during the Holocene [26] . Intervals of higher growth rates ( Fig. 3a ) coincide with some, but not all, intervals of significant power in the multi-decadal bands in the δ 18 O record ( Fig. 3b ). Such multi-decadal variability may in part be an artifact of aliasing short-term variations (such as an annual cycle) with a time-variable sampling interval [27] , but subannual resolution is only achieved in five short sections with a length of one to seven decades, within the resolution of our age model. We find little or no relation between intervals of significant multi-decadal variability in δ 13 C and changes in growth rate ( Fig. 3a ). Given that our sampling is in continuous-block averages, and that the growth of OCNM speleothems is biased towards one season, we expect that effects of digital aliasing are small. We extract the decadal (<100-year) variability from the isotope time series using Monte–Carlo Singular Spectrum Analysis [28] and estimate the amplitude modulation by smoothing between peak absolute values with a 300-year Gaussian window ( Fig. 3 ). Time-varying amplitudes of multi-decadal variability in δ 18 O and δ 13 C generally covary ( Fig. 3f ), with intervals of high-amplitude variability corresponding to those times when there is significant power in these periods in both records ( Fig. 3b ), suggesting coherent changes in temperature and precipitation on these time scales. Similar to the wavelet analysis, several intervals of higher variability appear to correspond in part with faster growth rates, which may reflect a common response to climate change or may represent a modulation of the amplitude recorded in the speleothem by growth-rate variations. Additional insight into these apparent modes of variability is provided by the Morlet cross-wavelet [29] , which identifies the phase between the δ 13 C and δ 18 O time series, helping to distinguish between a precipitation (rapidly responding, thus in phase with climate) versus biomass (slowly responding, thus lagging climate) influence on δ 13 C. Observed in-phase variations characterize the centennial bands ( Supplementary Fig. S2 ), indicating simultaneous changes in precipitation (and associated drip rate) and temperature, and point to a process involving changes in large-scale synoptic atmospheric circulation patterns, analogous to the PDO, that today give rise to similar climatologies over the US Pacific Northwest. In the millennial band, δ 13 C lags δ 18 O by several hundred years (mean phase of 42±10° s.d.) ( Supplementary Fig. S2 ), suggesting a larger control by slowly responding biomass on δ 13 C than by the direct and rapid effects of drip rate. Such a slow vegetation response is supported by pollen studies at nearby sites in the Klamath Mountains [15] and in the Coast and Cascade Ranges [9] showing that vegetation can lag long-term climate change by centuries to a millennium, and is consistent with estimates of the time constant for biomass changes relative to climate in an analogous Southern-Hemisphere setting [30] . Centennial and millennial variability in Holocene records has often been attributed to solar forcing [31] , [32] , [33] , [34] , [35] , but the mechanism(s) by which that weak forcing induces climate change remain unclear. Direct measurements of solar activity are only available for the last three decades, but changes in past solar variability have been inferred from the production rates of cosmogenic nuclides in the upper atmosphere ( 14 C measured in tree rings, and 10 Be from ice cores) [36] , [37] . The production rate of these nuclides is related mostly to the activity of the sun, but other factors such as changes in the Earth’s magnetic field, climate and in the carbon cycle can influence their production. However, the shared features of these proxies likely reflect some component of solar activity [38] . Some models predict a solar modulation of tropical Pacific ENSO variability in which an increase (decrease) in radiative forcing enhances (decreases) the thermal gradient between the eastern and western Pacific, causing easterly winds to intensify (weaken), further enhancing (decreasing) the gradient through the Bjerknes feedback. In these models this feedback mechanism results in a rapid (~10-year) switch to a more persistent ‘La Niña-like (El Niño-like)’ state of the tropical ocean [39] , [40] , [41] . A simplified model of the tropical Pacific atmosphere–ocean system forced by solar and orbital changes over the last 10 ka found significant enhancement of ENSO variability at periods similar to those (~500 and ~1,000 years) identified here [42] . Given modern tropical Pacific teleconnections to the US Pacific Northwest and the evidence of such influences in the past [43] , we consider potential relationships between our speleothem record and a Pacific response to solar forcing by comparing it to cosmogenic nuclide proxies ( 10 Be and 14 C) of solar activity ( Fig. 4 ). Acknowledging that the relationship may be nonlinear, and considering uncertainties in the speleothem age model, seven of the eight cold-wet events that punctuate the climate of the last 8 ka (events ‘b’–‘h’) correspond to times of high solar activity inferred by the nuclide proxies. The only misfit, a minor cold-wet interval (event ‘a’) centred near 1.2 ka, overlaps with an interval of low solar activity at 1 ka. The age-model uncertainty for this event, however, permits a small (200-year) adjustment in the age model that could align it with the 10 Be and 14 C records of high solar activity similar to the other events ( Fig. 4 ). 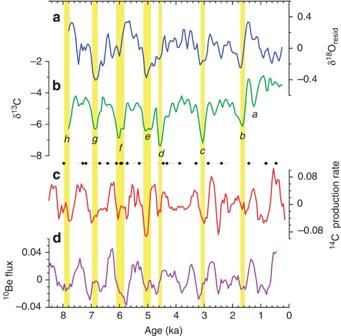Figure 4: OCNM stable isotopes and solar proxies. (a) Detrended δ18O time series at OCNM smoothed at 50-year resolution. (b) OCNM δ13C record smoothed at 50 years, with particularly pronounced negative excursions in the δ13C record identified as eventsa–h. Black diamonds below the δ13C time series represent the U-Th ages and associated 2σ uncertainties. (c) Estimated14C production rate37. (d) Estimated10Be flux in a Greenland ice core36. Both nuclide time series (c,d), inferred to reflect total solar irradiance, were filtered to remove periods >1,800 years and subdecadal noise35, then interpolated at 50-year resolution. Figure 4: OCNM stable isotopes and solar proxies. ( a ) Detrended δ 18 O time series at OCNM smoothed at 50-year resolution. ( b ) OCNM δ 13 C record smoothed at 50 years, with particularly pronounced negative excursions in the δ 13 C record identified as events a – h . Black diamonds below the δ 13 C time series represent the U-Th ages and associated 2σ uncertainties. ( c ) Estimated 14 C production rate [37] . ( d ) Estimated 10 Be flux in a Greenland ice core [36] . Both nuclide time series ( c , d ), inferred to reflect total solar irradiance, were filtered to remove periods >1,800 years and subdecadal noise [35] , then interpolated at 50-year resolution. Full size image An association of cold-wet events at OCNM with intervals of high solar activity is consistent with a reconstruction of early Holocene eastern tropical Pacific sea surface temperature (SST) variability ( Fig. 2e ), which found that cooler (La Niña-like) SSTs corresponded to high solar forcing during the early Holocene [35] ; in the higher resolution section of that study, the two youngest cold SST events (at ~7 and 7.8 ka) coincide with the two oldest cold-wet events in the OCNM record ( Fig. 4 ), and offer additional support for a teleconnected Pacific response at OCNM to solar forcing, mediated by ENSO [42] . The low resolution of the middle-to-late Holocene section of the tropical Pacific record ( Fig. 2e ) precluded an assessment of a continuation of solar forcing [35] , but our high-resolution OCNM record indicates that solar forcing may have influenced Pacific climate throughout the Holocene. In summary, our new high-resolution record from OCNM shows high variability of winter climate, including repeated abrupt (within decades) shifts between warm/dry and cool/wet conditions, which are plausibly linked to weak radiative forcing, perhaps via teleconnection to remote ENSO dynamics. Stable isotope and U-Th sampling We obtained the stable isotope profile for stalagmite OCNM02-1 by milling calcite powder continuously at 30 μm intervals. Stable isotopes were measured at Oregon State University on a Finnigan-MAT 252 mass spectrometer interfaced with a Kiel III online acid digestion device. Results are reported relative to the Vienna Pee Dee Belemnite (VPDB) standard and external precision on replicate samples (NBS 19, NBS 20, and a local carbonate standard) run daily on this system was 0.06‰ for δ 18 O and 0.02‰ for δ 13 C. This analytical noise floor, compared with power spectra of the data, shows that signal emerges consistently from noise at timescales of decades and longer. The raw and interpolated stable carbon and oxygen isotope values for stalagmite OCNM02-1 are provided in Supplementary Data 1 . An important first step in speleothem studies is to establish whether calcite was formed in isotopic equilibrium with cave dripwaters. Hendy [10] proposed two criteria to determine equilibrium fractionation of oxygen and carbon isotopes in speleothems: δ 18 O should be constant along a single growth layer and the covariance of δ 18 O and δ 13 C along the growth axis should be low. Although the latter criterion can be readily applied to speleothems, sampling along a single growth layer is difficult because of the slow speleothem growth rates, irregular layer shapes and thinning of the layers from the growth axis of the stalagmite towards the edges. We find that the longitudinal correlation between δ 18 O and δ 13 C is low for OCNM02-1 ( r 2 =0.13) and sampling along a growth layer in OCNM02-1 using a hand-held dental drill had nearly constant δ 18 O values (s.d.=0.06) ( Supplementary Fig. S3 ). We also sampled along a growth layer using a New Wave Micromill by first drilling a trench above the layer of interest and gradually milling in small increments until we reached the target layer. The samples collected away from the growth axis showed no systematic δ 18 O enrichment towards the edges of the stalagmite and had low δ 18 O variability (s.d.=0.04) ( Supplementary Fig. S3 ). Sample discontinuities and changes in growth axis required that the isotope sampling track be changed at six locations, 46.98, 49.5, 63.3, 64.2, 82.74, 83.58 mm (4.39, 4.65, 5.78, 5.81, 6.64, 6.68 ka) ( Supplementary Figs S1 and S4 , and marked in Fig. 3 ). Although great care was taken to assemble as continuous a time series as possible across these changes in the sampling track, some discontinuities in the time series, or uncertainties in the age scale, may occur at these points. The wavelet spectrum or filtered timeseries can be affected by any abrupt jumps in the timeseries at these points, for example as a scattering of frequencies from low to high frequencies. Such effects may be present at ~4.4, ~4.6, ~5.8 and ~6.7 ka ( Fig. 3b–g ). To minimize digital aliasing of the annual cycle in the unevenly spaced Holocene record, we interpolate to 4-year time steps, first by block-averaging in 1-year increments the few sections that have subannual resolution, and then using Gaussian interpolation with a smoothing window of 30 years (full width,±3σ). Occasional instrumental errors and sample discontinuities resulted in very short sections, where the resolution between consecutive samples is >20 years, and in one extreme instance at 82.9 mm the resolution between two consecutive samples is 50 years. The smoothing procedure effectively removes variance of less than a ~15-year period and, because multiple points are averaged, it reduces the average effective analytical error in the smoothed record by about a factor of four (that is, effective δ 18 O precision of 0.013‰, and effective δ 13 C precision of 0.005‰). Given unavoidable variations in the effective sampling interval associated with changing speleothem growth rates, some temporal variation in the noise floor is expected in the filtered results, because the number of samples within the filter window depend on the sampling interval. Growth rate may also affect the timeseries in some unexpected ways, considering that the full data variance includes signal (both deterministic and stochastic ‘red’ noise) and analytical ‘white’ noise. For purposes of time series analysis, the data are interpolated to constant time intervals with Gaussian smoothing. Because the depth spacing of samples is constant, where growth rate is high, the number of data points within the smoothing filter is larger, and by averaging the noise (and thus total amplitude) is reduced accordingly. Conversely, where the sample interval is lower, fewer data points are averaged within the filter window, and the noise amplitude is higher. Where growth rates are extremely low, sample time intervals are large (30–40 years, near 6.6 ka, and ~11 years from 7.5–8 ka) and decadal frequencies may be clipped (that is reduced) or aliased into lower frequencies. At the lower frequencies, where signal amplitudes are higher and sample intervals are adequate, such digital artifacts are not significant. Samples for U-Th dating were obtained by drilling ~200 mg of calcite powder parallel to the growth layers, which were processed following procedures described elsewhere [44] , [45] by using a multi-collector inductively coupled plasma mass spectrometry (Thermo-Scientific NEPTUNE) at the University of Minnesota. Speleothem grey scale We analysed the speleothem grey scale and found no correlation between grey scale and isotopes (the squared correlation coefficient for both grey scale versus δ 18 O and grey scale versus δ 13 C is <0.0001). The grey scale depth series were created from a high-resolution .tif image of the speleothem slab with the milling tracks, using NIH ImageJ software. The optical tracks were oriented parallel to the milling tracks, and as close as possible where the image did not visually show shadow or other edge effects. There was an unavoidable bright reflection, likely due to some surface roughness, near 50 mm. The width of the optical tracks was approximately the same as the width of the milled tracks. Five overlapping optical tracks were extracted from the image over the nominal depth ranges 0–50, 25–75, 60–80, 80–100 and 95–155 mm (note lack of overlap in the optical tracks at 80 mm, because it is difficult to visually follow the laminae at that jump in the milling track). These five intervals were then combined into a composite grey-scale depth series, working from the top down, with small adjustments to the nominal depths of each optical track defined at the splice points (46.5 66.5, 71.1, 80.0 and 98.1 mm), to align well-defined features. The final depth scale ( Supplementary Fig. S5 ) integrates all of these small depth adjustments. The nominal sampling increment (that is pixel resolution) in this composite depth series is 0.021 mm. This raw composite depth series was then interpolated to 0.03 mm intervals and filtered with a 0.09 mm Gaussian filter. There could be some small (sub-mm) depth mismatches between the composite grey scale depth series and the isotopic depth series, but shifting the grey scale data in one direction or another does not improve the correlation with either isotope record. Dripwater monitoring We monitored δ 18 O in cave dripwater over a period of three years, and we collected 179 water samples from four different locations, characterized by both slow drips and by fast fracture/conduit-type flow. The average δ 18 O value of these dripwaters is −11.3‰±0.9 s.d. ( Supplementary Table S2 ), which is similar to the average rainwater δ 18 O collected above the cave previously reported [4] (−11‰±4 s.d., n =48). This indicates that the cave dripwaters preserve the isotopic signature of rainwaters and the cave is effective in smoothing the intra-annual variability of rainwater δ 18 O. In addition, the two modern soda-straw stalactites collected in the cave have an average δ 18 O of −8.8‰, a value that falls between the calcite δ 18 O values predicted to form under equilibrium conditions at 7 °C from dripwaters at OCNM using the calcite-water fractionation factors of Coplen [46] (–8.56‰±0.96 s.d.) and Kim and O’Neil [47] (−9.9‰±0.94 s.d. ), although the most appropriate calcite-water fractionation factor for cave environments is still uncertain as it appears to change with both temperature and growth rate [48] . MCA versus LIA test The Shapiro–Wilk normality test [49] indicates that the OCNM data are not normally distributed ( P <0.05) and we therefore use the Mann–Whitney statistic [50] to evaluate the difference between δ 13 C values during the LIA and MCA. This difference is statistically significant, with median LIA and MCA values of −3.44‰ and −3.25‰, respectively ( U =2,654.5, n 1 =67, n 2 =100, P =0.023), and the lower LIA value is consistent with a wetter winter period. As a reference record, we combine the drought reconstruction from the three nearest grid points to our cave (033, 034 and 035) in The North American Drought Atlas [51] to obtain a composite drought record for our area. This tree-ring-derived drought reconstruction also suggests a wetter LIA compared with MCA (the median Pacific Drought Severity Index during MCA=−0.227 and during LIA=−0.138, Mann–Whitney- U =65,921, n 1 = n 2 =401, P <0.001). Thus, our results are consistent with the regional tree-ring records in suggesting a drier MCA and wetter LIA, but within each of these periods there is still significant variability. How to cite this article: Ersek V. et al. Holocene winter climate variability in mid-latitude western North America. Nat. Commun. 3:1219 doi: 10.1038/ncomms2222 (2012).